Dynamic blastomere behaviour reflects human embryo ploidy by the four-cell stage Previous studies have demonstrated that aneuploidy in human embryos is surprisingly frequent with 50–80% of cleavage-stage human embryos carrying an abnormal chromosome number. Here we combine non-invasive time-lapse imaging with karyotypic reconstruction of all blastomeres in four-cell human embryos to address the hypothesis that blastomere behaviour may reflect ploidy during the first two cleavage divisions. We demonstrate that precise cell cycle parameter timing is observed in all euploid embryos to the four-cell stage, whereas only 30% of aneuploid embryos exhibit parameter values within normal timing windows. Further, we observe that the generation of human embryonic aneuploidy is complex with contribution from chromosome-containing fragments/micronuclei that frequently emerge and may persist or become reabsorbed during interphase. These findings suggest that cell cycle and fragmentation parameters of individual blastomeres are diagnostic of ploidy, amenable to automated tracking algorithms, and likely of clinical relevance in reducing transfer of embryos prone to miscarriage. Efforts to elucidate key pathways of normal human embryo development and factors that contribute to embryo arrest and aneuploidy have benefited from recent advances in imaging, molecular and genetic analyses [1] , [2] , [3] , [4] , [5] . We previously used non-invasive time-lapse imaging to identify three dynamic cell cycle parameters that predict success or failure of human embryos to develop to the blastocyst stage, by the four-cell stage [1] . The three predictive parameters are duration of first cytokinesis, time from the two- to three-cell stage and synchronicity in appearance of the third and fourth blastomeres. Considering that the incidence of human embryonic aneuploidy is high (~50–80%) [5] and in light of the dynamic nature of the cell cycle parameters that predict successful development to the blastocyst stage, we contemplated whether non-invasive time-lapse imaging of dynamic human embryonic blastomere behaviour might provide a means to distinguish euploid from aneuploid embryos. In this study, we focused on correlating imaging and karyotypic data before embryonic genome activation in a unique set of embryos that were cryopreserved at the one-cell stage before assessment of quality and thus, likely to be representative of embryos typically obtained in the in vitro fertilization (IVF) clinic [1] , [6] , [7] , [8] . By correlating non-invasive time-lapse imaging with the chromosomal composition of all blastomeres in each human embryo, we demonstrate that cell cycle parameters in conjunction with dynamic fragmentation analysis largely reflect underlying ploidy to the four-cell stage. We also show that the high frequency of human embryonic aneuploidy, relative to other species [5] , [9] , [10] , has contributions from chromosome-containing fragments/micronuclei, which frequently arise during interphase and may have consequences for normal human development. Experimental design for assessing human blastomere behaviour The experimental design used to investigate the relationship between cell cycle parameters and ploidy is as shown ( Supplementary Fig. S1a ). Seventy-five human zygotes were cultured for 2 days and development was recorded to four cells by time-lapse imaging with image collection every 5 min. This experimental design allowed us to capture key cell cycle parameters and reconstruct embryo karyotypes, a task that is difficult given the complex aneuploidy and high rates of mosaicism in human blastomeres by the eight-cell stage [5] , [10] , [11] , [12] . Images from each experiment were then compiled into time-lapse movies and time intervals for each cell cycle parameter were measured manually by three independent evaluators ( Supplementary Fig. S1b,c ; Supplementary Movies 1 , 2 , 3 ). 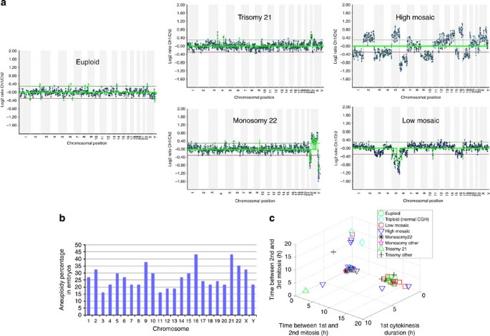Figure 1: Distinction between euploid and aneuploid embryos using dynamic parameter analysis. (a) A-CGH profiles of individual blastomeres showing the copy number of each chromosome in euploid, trisomy 21, monosomy 22, high-mosaic and low-mosaic embryos plotted in the 2D and 3D graphs. Copy number is based on the log2 ratio of the average signal intensity of the test to reference DNA for each chromosome. Low-mosaic embryos exhibited losses or gains in four chromosomes or less, whereas more than four chromosomes were affected in high-mosaic embryos. (b) Graphic representation of the incidence of aneuploidy observed in each chromosome for all human embryos used in the study and the surprisingly high frequency at which each chromosome is affected. (c) 3D plot displaying the correlation between the timing measurements of three parameters, the duration of the first cytokinesis, the interval between the first and second mitosis and the interval between the second and third mitosis and the underlying chromosomal composition of each imaged embryo. Embryos were categorized as euploid (green circles), triploid (aqua diamonds), low mosaic (red squares), high mosaic (downward pointing blue triangles), monosomy 22 (black asterisks), monosomy other (pink stars), trisomy 21 (upward pointing green triangles) and trisomy other (black plus signs) based on their A-CGH results. Note that all of the euploid embryos clustered together in a similar region as non-arrested or developmentally normal embryos in a previous report1, whereas aneuploid embryos either overlapped with euploid embryos or accumulated at or close to zero for the second cell cycle parameter;n=45. We observed that 53 of 75 embryos progressed beyond the zygote stage as is typical of human development ( Table 1 ). These embryos were disassembled for analysis of ploidy in each individual blastomere via 24-chromosome array-comparative genomic hybridization (A-CGH; Fig. 1a and Supplementary Fig. S1a ). Eight embryos were excluded for technical reasons such as cell lysis ( Table 1 ), resulting in analysis of 185 blastomeres from 45 embryos: 8 euploid, 34 aneuploid and 3 embryos, which appeared to be triploid ( Table 1 ), based on previous observations of a distinct morphological signature of dividing from a single cell to three daughter cells in the first cleavage division [1] . Our findings that ~75% of the human embryos analysed by A-CGH were aneuploid is consistent with previous studies [5] , [10] . We also determined that the high frequency of aneuploidy was not preferentially associated with a subset of chromosomes; instead, all 22 pairs of autosomes and both sex chromosomes were affected ( Fig. 1b ). Moreover, we also observed that in most cases (29 of 34), aneuploid embryos did not contain a single euploid blastomere capable of contributing to the embryo proper later in development ( Table 1 ). Table 1 Distinction between embryo ploidy states by A-CGH. Full size table Figure 1: Distinction between euploid and aneuploid embryos using dynamic parameter analysis. ( a ) A-CGH profiles of individual blastomeres showing the copy number of each chromosome in euploid, trisomy 21, monosomy 22, high-mosaic and low-mosaic embryos plotted in the 2D and 3D graphs. Copy number is based on the log2 ratio of the average signal intensity of the test to reference DNA for each chromosome. Low-mosaic embryos exhibited losses or gains in four chromosomes or less, whereas more than four chromosomes were affected in high-mosaic embryos. ( b ) Graphic representation of the incidence of aneuploidy observed in each chromosome for all human embryos used in the study and the surprisingly high frequency at which each chromosome is affected. ( c ) 3D plot displaying the correlation between the timing measurements of three parameters, the duration of the first cytokinesis, the interval between the first and second mitosis and the interval between the second and third mitosis and the underlying chromosomal composition of each imaged embryo. Embryos were categorized as euploid (green circles), triploid (aqua diamonds), low mosaic (red squares), high mosaic (downward pointing blue triangles), monosomy 22 (black asterisks), monosomy other (pink stars), trisomy 21 (upward pointing green triangles) and trisomy other (black plus signs) based on their A-CGH results. Note that all of the euploid embryos clustered together in a similar region as non-arrested or developmentally normal embryos in a previous report [1] , whereas aneuploid embryos either overlapped with euploid embryos or accumulated at or close to zero for the second cell cycle parameter; n =45. Full size image Detection of meiotic and mitotic errors by the four-cell stage On the basis of the results of chromosome analysis, we next sought to differentiate between types of errors in each aneuploid embryo. For this purpose, we inferred that aneuploid 4-cell embryos that were: (1) characterized by different chromosome compositions between blastomeres had incurred mitotic errors and (2) those with identical aneuploidies in all four blastomeres had most likely inherited meiotic errors. Thus, we concluded that 20% of 4-cell embryos (9/45) exhibited meiotic errors and >50% of the embryos (25/45) displayed mitotic errors, suggesting that the generation of chromosomal errors during the four-cell stage is most frequently mitotic in origin ( Table 1 ). Of the nine embryos with meiotic errors, we identified two embryos with trisomy 21, one of the most common types of autosomal trisomy that survives to birth, resulting in Down syndrome, and three embryos with monosomy 22, which is incompatible with live birth ( Fig. 1a ). In embryos with mitotic errors, while we observed simple mitotic mosaicism in which the same single chromosome was affected in the blastomeres of some embryos, the majority (20/25) of embryos exhibited complex mosaicism, or an abnormal number of multiple chromosomes within one or more blastomeres of an embryo ( Table 1 ). Cell cycle parameter timing in euploid and aneuploid embryos Next, we examined the mean values and s.d. of cell cycle parameters in embryos that were determined to be chromosomally normal. We observed complete overlap with previous reports [1] but with smaller s.d. : (i) 14.4±4.2 min duration of the first cytokinesis from the first cleavage furrow to the appearance of two distinct blastomeres, (ii) 11.8±0.71 h from two cells to the appearance of a third cell, and (iii) 0.96±0.84 h time from three to four cells ( Supplementary Table S1 ). In contrast, embryos with meiotic errors exhibited a much greater s.d. than euploid embryos in all three parameters ( n =9, *= P <0.05 by analysis of variance (ANOVA); P =0.06 by Kruskal–Wallis), including the duration of the first cytokinesis. Further, a higher s.d. in the time interval from two to three cells and the synchronicity in the appearance of the third and fourth cells ( n =25, *= P <0.05 by ANOVA; P =0.08 by Kruskal–Wallis) was observed in embryos with mitotic errors ( Supplementary Table S1 ), especially those with high mitotic mosacism ( n =13, **= P <0.01 by ANOVA; *= P <0.05 by Kruskal–Wallis). The calculated sensitivity and specificity of the parameters when used to predict euploidy by Fisher’s exact test was 100% and 66%, respectively, given that all embryos predicted to be aneuploid by imaging behaviour were actually chromosomally abnormal ( n =45, P <0.001). We next graphed each embryo as a point in a three-dimensional (3D) plot, where each dimension represented a cell cycle parameter. Embryos with normal karyotypes clustered together in a region nearly identical to non-arrested or developmentally normal embryos as previously observed [1] ( Fig. 1c ). In contrast, ~70% of the aneuploid embryos exhibited parameter values outside the timing windows of euploid embryos and, therefore, concentrated in other areas away from the euploid embryo clustering when graphed. Although 11 of 25 embryos with mitotic errors concentrated in a similar two- and 3D area as embryos with normal A-CGH profiles, the set of embryos with meiotic errors exhibited more sporadic parameter clustering in plots ( Fig. 1c and Supplementary Fig. S2a–c ). Embryos that appeared to be triploid ( Table 1 ), on the other hand, accumulated close to zero for the second parameter in 3D plots [1] ( Fig. 1c ). We verified triploidy via fluorescent in situ hybridization (FISH) of chromosome 18 in a single blastomere of an embryo that appeared to be triploid during time-lapse imaging analysis ( Supplementary Fig. S3a,b ). This observation further indicated that alterations in ploidy are reflected in cell cycle parameters of developing human embryos. Distinction between low/high-degree mitotic mosaicism Given the overlap in parameters of a subset of embryos with mitotic errors with those of euploid embryos ( Supplementary Fig. S2b ), we further examined the relationship between chromosomal composition of each blastomere and cell cycle characteristics. Embryos that had blastomeres with a low degree of mitotic mosaicism were associated with tighter clustering of cell cycle parameters near euploid embryos; a shift in parameter timing appeared to occur when four or fewer chromosomes were segregated abnormally ( Fig. 1c , Supplementary Fig. S2d and Supplementary Table S2 ). Thus, we classified embryos with defects in four chromosomes or fewer as ‘low mosaic’ and designated embryos with more than four chromosomes affected as ‘high mosaic’ ( Fig. 1a ). The term ‘mosaic’ is used here to refer to the presence of multiple aneuploidies within a single blastomere rather than mosaicism between blastomeres. Individual parameter analysis revealed that although low mosaic embryos had cell cycles more similar to embryos with normal karyotypes, high mosaic embryos deviated significantly, particularly in the time between the first and second mitosis ( Supplementary Table S1 ). Of the embryos with mitotic errors, we also determined that eight, in addition to two triploid embryos, had subchromosomal losses and/or gains, most of which were unbalanced ( Supplementary Table S3 and Supplementary Fig. S4 ). Thus, our findings to this point indicated differences in cell cycle parameters associated with the generation of different types of chromosomal abnormalities, including partial chromosome losses and/or gains. Correlation between cellular fragmentation and aneuploidy Under current clinical IVF practice, developmental competence of human embryos is assessed most commonly on day 3 or day 5 of culture based on morphological characteristics that may include blastomere number, blastomere symmetry and the degree of cellular fragmentation [13] , [14] , [15] , [16] . Cellular fragmentation, or the generation of what is commonly thought to be cytoplasmic fragments, occurs frequently in human embryos [13] , and is distinct from DNA fragmentation associated with cell death late in preimplantation development [17] , [18] . There is evidence to suggest that embryo fragmentation occurs in vivo , not just in vitro [19] , [20] , and that it may be negatively correlated with implantation potential [14] , [21] . In examining time-lapse images and dynamic behaviours of human embryos, we observed that a large proportion of aneuploid and triploid, but not euploid embryos, exhibited cellular fragmentation ( Supplementary Table S4 ). When we analysed cell cycle imaging parameters in embryos that did and did not exhibit fragmentation ( Fig. 2a ), we determined that dynamic assessment of fragmentation might assist in distinguishing euploid and aneuploid embryos with parameters that clustered together ( Fig. 2b ). However, only 65% of the embryos characterized by the presence of fragments would be predicted to form blastocysts ( Fig. 2c ), a value in accordance with the findings of Wong et al [1] . In addition, fragmentation screening in the absence of other morphological and/or dynamic criteria had minimal effect on the probability of embryonic euploidy in comparison with inclusion of analysis of cell cycle parameters ( Supplementary Fig. S5 and Supplementary Table S5 ). This was exemplified by calculating the probability of embryonic euploidy versus aneuploidy using fragmentation and/or parameter screening criteria if 1, 2 or 3 embryos were selected ( Supplementary Fig. S6 and Supplementary Table S6 ). 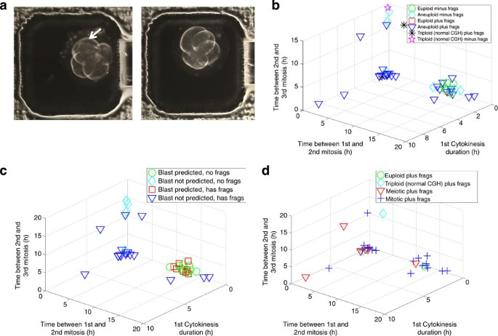Figure 2: Association between embryonic aneuploidy and cellular fragmentation. (a) The last frame of a time-lapse imaging sequence taken from an embryo with (left—indicated by white arrow) and without (right) fragmentation corresponding to the chromosomal composition outlined inSupplementary Table S2a and S2b, respectively. (b) Euploid embryos with (red squares) and without (green circles) fragmentation, aneuploid embryos with (blue triangles) and without (aqua diamonds) fragmentation and triploid embryos with (black asterisks) and without (pink stars) fragmentation were graphed in a 3D plot. Although fragmentation was detected in only one euploid embryo, the majority of both aneuploid and triploid embryos exhibited fragmentation;n=45. (c) Substantial overlap between embryos predicted to form blastocysts that do or do not exhibit fragmentation as illustrated in a 3D plot of blastocyst prediction with (red squares) and without (green circles) fragments (frags) and no blastocyst prediction with (blue triangles) and without (aqua diamonds) fragmentation. (d) A 3D plot demonstrating that in contrast to triploid embryos with fragmentation (aqua diamonds) and those with meiotic errors and fragmentation (red triangles), with the exception of one embryo with a meiotic error, only embryos with mitotic errors and fragmentation (blue plus signs) cluster near euploid embryos (green circles);n=32. Figure 2: Association between embryonic aneuploidy and cellular fragmentation. ( a ) The last frame of a time-lapse imaging sequence taken from an embryo with (left—indicated by white arrow) and without (right) fragmentation corresponding to the chromosomal composition outlined in Supplementary Table S2a and S2b , respectively. ( b ) Euploid embryos with (red squares) and without (green circles) fragmentation, aneuploid embryos with (blue triangles) and without (aqua diamonds) fragmentation and triploid embryos with (black asterisks) and without (pink stars) fragmentation were graphed in a 3D plot. Although fragmentation was detected in only one euploid embryo, the majority of both aneuploid and triploid embryos exhibited fragmentation; n =45. ( c ) Substantial overlap between embryos predicted to form blastocysts that do or do not exhibit fragmentation as illustrated in a 3D plot of blastocyst prediction with (red squares) and without (green circles) fragments (frags) and no blastocyst prediction with (blue triangles) and without (aqua diamonds) fragmentation. ( d ) A 3D plot demonstrating that in contrast to triploid embryos with fragmentation (aqua diamonds) and those with meiotic errors and fragmentation (red triangles), with the exception of one embryo with a meiotic error, only embryos with mitotic errors and fragmentation (blue plus signs) cluster near euploid embryos (green circles); n =32. Full size image We next focused our analysis on the embryos that exhibited fragmentation and determined the number of embryos with underlying meiotic and mitotic errors, high and low mosaicism, subchromosomal errors and those that appeared to be triploid ( Fig. 2d , Supplementary Fig. S7a and Supplementary Table S4 ). We observed that all of the aneuploid embryos with additional unbalanced subchromosomal errors exhibited fragmentation, whereas the one embryo with a balanced translocation between two blastomeres did not ( Supplementary Table S3 ). Moreover, we determined that additional fragmentation criteria such as the degree and developmental timing of cellular fragmentation or the inclusion of blastomere asymmetry in combination with cell cycle parameter analysis might also aid in embryo assessment ( Supplementary Fig. S7b and Supplementary Fig. S7c ). These findings suggest that although fragmentation alone is not able to predict developmental potential in embryos, especially when it is assessed at a single time point as is common in IVF clinics, time-lapse imaging in conjunction with dynamic fragmentation screening may aid in detecting embryonic aneuploidies of diverse origins. Containment of chromosomes within fragments During the course of these studies, we observed that individual blastomeres of aneuploid embryos often exhibited either chromosomal losses or gains, the sum of which did not always add-up to two copies of each chromosome per blastomere in each embryo ( Supplementary Table S2 ). More detailed analysis of chromosome composition also revealed complex genotypes in some embryos that were not in agreement with the typical 3:1 chromosomal ratios detected following mitotic non-disjunction even though A-CGH has been validated repeatedly and probe selection provides redundant coverage of all human chromosomes [22] ( Supplementary Table S2 ). Thus, given the observation that aneuploid embryos appeared to be associated with fragmentation ( Fig. 2 ), we explored whether missing chromosomes may have been sequestered into fragments during development. Indeed, we determined that fragmentation was observed in the majority of embryos (11 of 14) that did not have the correct total number of copies of a given chromosome ( Fig. 3a ). We suspect that the lack of observed fragmentation in the three embryos that displayed the incorrect chromosome copy number may be explained by the previous finding that some fragments may not be easily detected by light microscopy, including time-lapse microscopic imaging, but can be recognized at a higher magnification using alternative optics [13] . 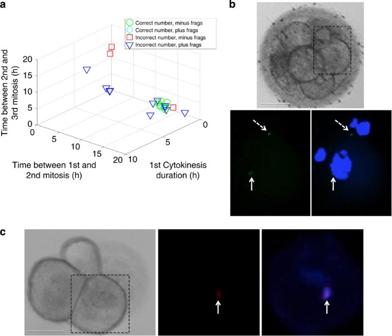Figure 3: Evidence for the sequestering of chromosomes within cellular fragments. (a) 3D plot showing the relationship between correct chromosome copy number defined as two copies of each chromosome per blastomere minus fragmentation (frags; green circles) or plus fragmentation (aqua diamonds) and incorrect chromosome copy number minus fragmentation (red squares) or plus fragmentation (blue triangles). Note that fragmentation may be used to identify embryos with abnormal chromosome number(s) that exhibit normal parameter timing;n=23. (b) FISH analysis of a single blastomere shown by the dashed box from a cleavage-stage embryo exhibiting cellular fragmentation and visualized by DIC (top) and confocal microscopy (bottom left and right). Two FISH signals for chromosome 16 were detected in the primary nucleus of the blastomere (bottom left; indicated by white solid arrow) stained with DAPI in the merged image (bottom right), but also one chromosome 16 signal was observed outside the primary nucleus of the blastomere (shown by white dashed arrow). (c) Similar FISH analysis of an individual blastomere indicated by the dashed box from an embryo without fragmentation (left) showing 1–2 copies of chromosome 21 (middle) in a small nuclear structure distinct from the primary nucleus of the blastomere (right). Scale bar, 50 μm. Figure 3: Evidence for the sequestering of chromosomes within cellular fragments. ( a ) 3D plot showing the relationship between correct chromosome copy number defined as two copies of each chromosome per blastomere minus fragmentation (frags; green circles) or plus fragmentation (aqua diamonds) and incorrect chromosome copy number minus fragmentation (red squares) or plus fragmentation (blue triangles). Note that fragmentation may be used to identify embryos with abnormal chromosome number(s) that exhibit normal parameter timing; n =23. ( b ) FISH analysis of a single blastomere shown by the dashed box from a cleavage-stage embryo exhibiting cellular fragmentation and visualized by DIC (top) and confocal microscopy (bottom left and right). Two FISH signals for chromosome 16 were detected in the primary nucleus of the blastomere (bottom left; indicated by white solid arrow) stained with DAPI in the merged image (bottom right), but also one chromosome 16 signal was observed outside the primary nucleus of the blastomere (shown by white dashed arrow). ( c ) Similar FISH analysis of an individual blastomere indicated by the dashed box from an embryo without fragmentation (left) showing 1–2 copies of chromosome 21 (middle) in a small nuclear structure distinct from the primary nucleus of the blastomere (right). Scale bar, 50 μm. Full size image To further test whether fragments may contain missing chromosomes, we stained zona pellucida (ZP)-free cleavage-stage human embryos with the nucleic acid dye, DAPI (4′,6-diamidino-2-phenylindole). As shown by confocal imaging ( Supplementary Fig. S8a ) and 3D modelling ( Supplementary Fig. S8b,c ), we observed localization of DNA within fragments (indicated by white arrow in DAPI images and solid black arrow in differential interference contrast (DIC)/merged images). We also observed fragments negative for DAPI staining (shown by dashed black arrow) adjacent to DAPI-positive fragments, indicating that some but not all fragments contain nuclear DNA and eliminating the possibility that these fragments were polar bodies, which should have degenerated or initiated degeneration by this stage of development [23] ( Supplementary Fig. S8a ). These findings were supported by DNA–FISH for some of the most commonly affected chromosomes in human embryonic development [24] in single blastomeres from dissembled embryos. Although we observed two copies of chromosome 16 in the primary nucleus of a blastomere from a fragmented embryo (indicated by white solid arrow; Fig. 3b ), an additional chromosome 16 FISH signal also appeared separate from the primary nucleus (shown by white dashed arrow; Fig. 3b ). In another example, we detected one to two copies of chromosome 21 (indicated by white solid arrow; Fig. 3c ) in a smaller nuclear structure distinct from the primary nucleus of a blastomere taken from an embryo that did not exhibit fragmentation. Chromosome-containing fragments may arise from micronuclei As further evidence of chromosome sequestering within fragments, we immunostained cleavage-stage human embryos with the centromeric marker, centromere protein-A (CENP-A) and the nuclear envelope marker, LAMIN-B1. Not only did we observe positive CENP-A expression in LAMIN-B1 encapsulated nuclei of blastomeres, but we also detected CENP-A immunosignals indicative of multiple missing chromosomes in cellular fragments as well (indicated by white arrows; Fig. 4a and Supplementary Fig. S9a,b ). Notably, CENP-A expression was also observed in small structures enveloped by LAMIN-B1 expression ( Fig. 4a and Supplementary Fig. S9a,b ) that resembled those detected by DNA–FISH ( Fig. 3c ). We termed these structures embryonic micronuclei and based on their distinct expression pattern, suggest that missing chromosomes are encapsulated in micronuclei before being sequestered into fragments (shown by white arrows; Fig. 4a and Supplementary Fig. S9a,b ). In contrast, cleavage-stage mouse embryos typically only exhibit Lamin-B1 expression around the primary nucleus of each blastomere ( Fig. 4b and Supplementary Fig. S9c ). We also found that encapsulated micronuclei were observed in >50% (13 out of 25) of cleaving human embryos, concordant with the percentage of mitotic chromosomal errors detected in this study ( Table 1 and Supplementary Fig. S2a,b ). 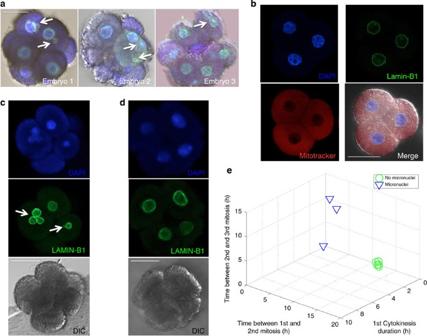Figure 4: Detection and developmental consequences of embryonic micronuclei. (a) LAMIN-B1 (green) and CENP-A (orange) expression in DAPI-stained (blue) cleavage-stage human embryos by confocal microscopy reveals chromosome-containing micronuclei in the blastomeres of human embryos (shown by white arrows), (b) but not in mouse embryos also stained with Mitotracker Red. (c) Detection of embryonic micronuclei by LAMIN-B1 immunostaining in human embryos with abnormal cell cycle parameters, (d) but not in those with normal parameter timing. (e) 3D plot showing the effects of micronuclei on the cell cycle parameters and embryo developmental potential. Note that embryos without micronuclei (green circles) tightly cluster in a region similar to embryos with normal A-CGH profiles, whereas those embryos with micronuclei (blue triangles) exhibit more diverse parameter clustering when graphed;n=8. Scale bar, 50 μm. Figure 4: Detection and developmental consequences of embryonic micronuclei. ( a ) LAMIN-B1 (green) and CENP-A (orange) expression in DAPI-stained (blue) cleavage-stage human embryos by confocal microscopy reveals chromosome-containing micronuclei in the blastomeres of human embryos (shown by white arrows), ( b ) but not in mouse embryos also stained with Mitotracker Red. ( c ) Detection of embryonic micronuclei by LAMIN-B1 immunostaining in human embryos with abnormal cell cycle parameters, ( d ) but not in those with normal parameter timing. ( e ) 3D plot showing the effects of micronuclei on the cell cycle parameters and embryo developmental potential. Note that embryos without micronuclei (green circles) tightly cluster in a region similar to embryos with normal A-CGH profiles, whereas those embryos with micronuclei (blue triangles) exhibit more diverse parameter clustering when graphed; n =8. Scale bar, 50 μm. Full size image To determine whether the appearance of embryonic micronuclei had any effects on developmental potential, we cultured an additional set of human embryos from the zygote to approximately the four-cell stage and monitored embryonic development by time-lapse imaging. Once the cell cycle parameter values were determined for each embryo, we immunostained for LAMIN-B1; blinded results were then scored for normal and abnormal parameter timing. Although LAMIN-B1 expression was confined to the primary nucleus of each blastomere in embryos with normal parameter timing windows, multiple LAMIN-B1-encapsulated micronuclei were detected in one or more embryonic blastomeres of all embryos with abnormal parameter timing ( Fig. 4c and Supplementary Fig. S10 ). When each embryo was graphed as a point in a 3D parameter plot, the embryos without micronuclei concentrated in a similar 3D area as embryos with normal A-CGH profiles, whereas the embryos with micronuclei exhibited more sporadic parameter clustering ( Fig. 4e ). Thus, contrary to notions that chromosomal errors are only due to meiotic or mitotic non-disjunction, which manifests as the chromosomes are congressing and then segregating from one another on the spindle [25] , our analysis suggests that there may be a contribution to aneuploidy arising from fragmentation of blastomeres carrying human chromosomes. Proposed model of aneuploidy generation in human embryos Our time-lapse image analysis suggested that as development proceeds, embryonic fragments may remain as separate units that carry chromosomal DNA and cytoplasm, or alternatively, fragments may also be reabsorbed by the same blastomere from which they were produced or fuse with a neighbouring blastomere(s) ( Fig. 5a and Supplementary Movies 4 ) as previously suggested [26] , [27] , [28] . If a chromosome-containing fragment fuses with the blastomere from which it originated, it could potentially restore embryonic euploidy following nuclear envelope breakdown ( Fig. 5c ), which may explain the single euploid embryo with fragmentation observed in this study ( Fig. 2b ) and also previous findings of occasional chromosomal correction during embryo development [29] , [30] . However, equally likely is the fusion of a fragment with sequestered chromosome(s) to a neighbouring blastomere ( Fig. 5c ), resulting in the complex genotypes observed in this study ( Supplementary Table S2 ) and others [5] , [10] . 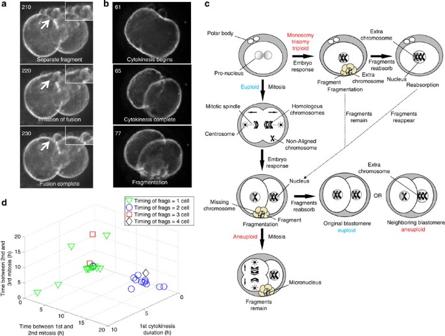Figure 5: Fragmentation timing suggests an embryo response to chromosomal abnormalities. (a) Individual frames indicated by numbers taken from a time-lapse imaging sequence (Supplementary Movie 4) of an embryo with fragmentation demonstrating the fusion of a cellular fragment with an embryonic blastomere, which helps explain the complexity and incongruence of aneuploidy detected in human embryonic blastomeres. (b) Numbered imaging frames fromSupplementary Movie 6showing the incidence of cellular fragmentation following completion of the first cytokinesis. (c) Proposed model for the origin of human embryonic aneuploidy based on fragmentation timing, fragment resorption and underlying chromosomal abnormalities. Human embryos with meiotic errors (monosomies and trisomies) and those that appear to be triploid typically exhibit fragmentation at the one-cell stage (Supplementary Movie 5), whereas fragmentation is most often detected at the two-cell stage in embryos with mitotic errors (Supplementary Movie 6). We also demonstrate that missing chromosome(s) are contained within fragments (Supplementary Fig. S9a) termed embryonic micronuclei and for those embryos with mitotic errors, propose that the embryo likely divided before these chromosomes properly aligned on the mitotic spindle. The correlation between the timing of fragmentation and the type of embryonic aneuploidy suggests that the embryo may respond to chromosomal abnormalities and undergoes fragmentation as a survival mechanism. As development proceeds, these fragments either remain or are reabsorbed by the blastomere from which they originated or a neighbouring blastomere to generate the complex human aneuploidies observed (Supplementary Movie 4). (d) 3D plot showing the relationship between the timing of fragmentation and the cell cycle imaging parameters. Note that fragmentation, which is observed at the one-cell stage or later in development at the three to four-cell stage has more detrimental effects on the imaging parameters than fragmentation that occurs at the two-cell stage;n=32. Figure 5: Fragmentation timing suggests an embryo response to chromosomal abnormalities. ( a ) Individual frames indicated by numbers taken from a time-lapse imaging sequence ( Supplementary Movie 4 ) of an embryo with fragmentation demonstrating the fusion of a cellular fragment with an embryonic blastomere, which helps explain the complexity and incongruence of aneuploidy detected in human embryonic blastomeres. ( b ) Numbered imaging frames from Supplementary Movie 6 showing the incidence of cellular fragmentation following completion of the first cytokinesis. ( c ) Proposed model for the origin of human embryonic aneuploidy based on fragmentation timing, fragment resorption and underlying chromosomal abnormalities. Human embryos with meiotic errors (monosomies and trisomies) and those that appear to be triploid typically exhibit fragmentation at the one-cell stage ( Supplementary Movie 5 ), whereas fragmentation is most often detected at the two-cell stage in embryos with mitotic errors ( Supplementary Movie 6 ). We also demonstrate that missing chromosome(s) are contained within fragments ( Supplementary Fig. S9a ) termed embryonic micronuclei and for those embryos with mitotic errors, propose that the embryo likely divided before these chromosomes properly aligned on the mitotic spindle. The correlation between the timing of fragmentation and the type of embryonic aneuploidy suggests that the embryo may respond to chromosomal abnormalities and undergoes fragmentation as a survival mechanism. As development proceeds, these fragments either remain or are reabsorbed by the blastomere from which they originated or a neighbouring blastomere to generate the complex human aneuploidies observed ( Supplementary Movie 4 ). ( d ) 3D plot showing the relationship between the timing of fragmentation and the cell cycle imaging parameters. Note that fragmentation, which is observed at the one-cell stage or later in development at the three to four-cell stage has more detrimental effects on the imaging parameters than fragmentation that occurs at the two-cell stage; n =32. Full size image After further evaluating the correlation between timing of fragmentation and cell cycle imaging parameters, we observed that the most significant effects on parameter windows were observed in embryos in which fragmentation occurred either at the one-cell stage or to a lesser extent at the three- to four-cell stage ( Fig. 5d ). Following analysis of embryonic chromosomal composition, we determined that embryos with meiotic errors or those that appeared to be triploid by imaging consistently exhibited fragmentation at the one-cell stage before the first cytokinesis ( Supplementary Table S4 and Supplementary Movies 5 ). In contrast, fragmentation was typically observed later, following the division of one to two cells in embryos with mitotic errors ( Supplementary Table S4 ) and also often during interphase, or following the completion of the first cytokinesis ( Fig. 5b and Supplementary Movie 6 ). It is important to note that the blastomeres of the embryos with mitotic errors, which began fragmenting at the one-cell stage ( Supplementary Table S4 ), also exhibited complex mitotic mosaicism with multiple missing chromosomes, indicating that these embryos may have inherited a meiotic error followed by generation of a mitotic error. For those embryos with mitotic errors, we also propose in our model that these embryos likely divided before all the chromosomes had a chance to properly align on the mitotic spindle ( Fig. 5c ), which is supported by findings of lagging chromosomes during anaphase in human embryos [31] . Whether the generation of micronuclei and cellular fragmentation represents a potential means to correct the embryonic aneuploidy ( Fig. 5c ) or is the initiation of eventual demise later in development [17] , [18] remains to be determined. The generation of aneuploidy in human embryos, as defined here, precedes the major wave of embryonic genome activation that occurs at approximately the eight-cell stage [1] , [2] , [3] , [4] , [5] , [6] , [7] . Thus, the human embryo has limited ability to respond with a transcriptional cascade that could culminate with apoptosis, but must rely on translational programs. Automated tracking of cumulative fragmentation As evidenced by our time-lapse image analysis of early human embryo development, manual characterization of certain developmental events, such as fragmentation, is subject to interpretation and timing of observations. To minimize variability in interpretation and account for changes in fragmentation patterns over time, we sought to develop an automated fragmentation detector to systematically quantify the cumulative degree of fragmentation, independent of whether fragment reabsorption had occurred, and validate our manual fragmentation measurements. We performed automated fragmentation analysis on the sixteen embryos shown in Supplementary Movie 1 and overlaid the segment detection to produce the composite video in Supplementary Movie 7 . By graphing the cumulative length of fragment segments over time for each embryo, we observed a clear correlation between combined segment length and degree of fragmentation as shown by three representative cases of embryos with high, low or no fragmentation ( Fig. 6a ). We defined the fragmentation score of each embryo to be the cumulative segment length for all imaging frames and used this score for comparison with our manual measurements of fragmentation degree. Although we detected partial overlap in the fragmentation score of embryos with no or low fragmentation, there was strong agreement between the fragmentation scores obtained by automated fragment detection and our manual fragmentation measurements ( Fig. 6b ). Thus, these results indicate that computer-assisted automated image analysis can provide a quantitative, objective and reliable measure of fragmentation over time for additional large sets of imaging data and in statistical fragmentation studies of patient embryos ( Figs 6c and 7 ). 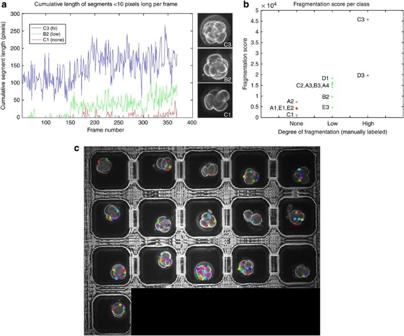Figure 6: Automated tracking of cellular fragmentation for embryo assessment. (a) Time sequence of cumulative segment lengths in pixels for each frame of the time-lapse image analysis for embryo C3 with high fragmentation, embryo B2 with low fragmentation and embryo C1 with no fragmentation shown inSupplementary Movie 1. Note that the embryo with high fragmentation exhibits much larger cumulative length of segments than that of embryos with low or no fragmentation. The alphanumeric labels of these embryos refer to the corresponding microwell identification labels. (b) Scatter plot of fragmentation scores for 14 of the 16 embryos (two embryos were excluded from the analysis for technical reasons) shown inSupplementary Movie 7based on manual measurement of fragmentation degree. The fragmentation score is the cumulative sum of all segment lengths <10 pixels across all imaging sequences of each embryo. Although there is partial overlap in the fragmentation score between embryos with no or low fragmentation, the automated fragmentation detector validates the degree of the fragmentation measured manually. (c) The last frame of an image sequence compiled into a time-lapse movie (Supplementary Movie 7) overlaid with the automatic fragmentation analysis. Figure 6: Automated tracking of cellular fragmentation for embryo assessment. ( a ) Time sequence of cumulative segment lengths in pixels for each frame of the time-lapse image analysis for embryo C3 with high fragmentation, embryo B2 with low fragmentation and embryo C1 with no fragmentation shown in Supplementary Movie 1 . Note that the embryo with high fragmentation exhibits much larger cumulative length of segments than that of embryos with low or no fragmentation. The alphanumeric labels of these embryos refer to the corresponding microwell identification labels. ( b ) Scatter plot of fragmentation scores for 14 of the 16 embryos (two embryos were excluded from the analysis for technical reasons) shown in Supplementary Movie 7 based on manual measurement of fragmentation degree. The fragmentation score is the cumulative sum of all segment lengths <10 pixels across all imaging sequences of each embryo. Although there is partial overlap in the fragmentation score between embryos with no or low fragmentation, the automated fragmentation detector validates the degree of the fragmentation measured manually. ( c ) The last frame of an image sequence compiled into a time-lapse movie ( Supplementary Movie 7 ) overlaid with the automatic fragmentation analysis. 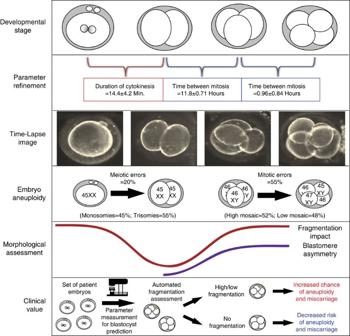Figure 7: Summary model of human embryonic aneuploidy. Embryonic development was monitored by time-lapse imaging from the one- to four-cell stage followed by assessment of chromosomal composition of each blastomere in the imaged embryos. We observed refinement of diagnostic non-invasive cell cycle parameters, determined the correlation with meiotic (monosomies and trisomies) and mitotic (high and low mosaic) errors and demonstrated an association between the cell cycle parameters and embryo morphology (fragmentation and blastomere asymmetry). We also suggest clinical value of parameter analysis with and without automated fragmentation assessment. Full size image Figure 7: Summary model of human embryonic aneuploidy. Embryonic development was monitored by time-lapse imaging from the one- to four-cell stage followed by assessment of chromosomal composition of each blastomere in the imaged embryos. We observed refinement of diagnostic non-invasive cell cycle parameters, determined the correlation with meiotic (monosomies and trisomies) and mitotic (high and low mosaic) errors and demonstrated an association between the cell cycle parameters and embryo morphology (fragmentation and blastomere asymmetry). We also suggest clinical value of parameter analysis with and without automated fragmentation assessment. Full size image Over the past few decades, elegant studies in model systems including yeast, flies, worms, fish and frogs have compared chromosome dynamics in wildtype and mutant cells that display diverse phenotypes [32] , [33] , [34] , [35] , [36] , [37] , [38] , [39] . Particularly in Caenorhabditis elegans , studies of mutations in genes that affect the first embryonic cell divisions are enlightening. For example, in 1994 Gonczy et al . [37] reported a collection of 48 maternal-effect embryonic lethal mutations on chromosome III that they characterized phenotypically by time-lapse DIC video microscopy. The mutations mapped to 34 loci and were characterized by defects in pronuclear migration, rotation of centrosomes and associated pronuclei, spindle assembly, chromosome segregation, anaphase spindle positioning and cytokinesis. Subsequent studies have examined the molecular mechanisms that underlie these phenotypic classes and others [32] , [33] , [40] , [41] . In other species such as the zebrafish, Danio Rerio , and the frog, Xenopus laevis, karyomeres form to accommodate the large cells formed following fertilization [38] , [39] . Karyomeres are thought to provide mitotic intermediates that are comprised of chromatin masses surrounded by nuclear envelope, which then fuse to form a single nucleus as recently described in more detail by Mullins and colleagues [38] . When we compare these studies to our data, we observe that a subset of images from these organisms clearly resemble those we observed with formation of multiple micronuclei in human embryos. This suggests the possibility that embryonic micronuclei observed in human embryos may be formed via conserved pathways that allow encapsulation of chromosomes in nuclear envelope either under normal developmental conditions or in response to chromosome detachment from the spindle during cleavage divisions. In this study, we observed that chromosomally normal embryos display strict and tightly clustered cell cycle parameters, whereas chromosomally abnormal embryos exhibit more diverse parameters that may or may not overlap those of euploid embryos. By the four-cell stage of development, we observed that dynamic assessment of cell cycle parameters in conjunction with fragmentation analysis and blastomere asymmetry assists in the differentiation between the type of error (meiotic versus mitotic), detects chromosomal duplications (trisomies) and deletions (monosomies) and provides a reliable readout of the degree of mitotic mosaicism (high versus low) in human embryos. Furthermore, we observed that the generation of partial chromosomal gains and losses was restricted primarily to embryos with mitotic errors, suggesting a relationship between subchromosomal instability and aneuploidy in the human embryo. We also demonstrate that human embryonic aneuploidy and mosaicism of chromosome content between blastomeres [5] , [10] , [11] , [12] may have contributions from a phenomenon that encompasses the formation of embryonic micronuclei, cellular fragmentation and resorption. Thus, practices that were once promoted such as embryo surgery for the removal of fragments are likely to result in the removal of micronuclei and perhaps genetic information and may potentially be deleterious [42] , [43] . On the basis of the timing of fragmentation and our time-lapse image analysis, we suggest that the human embryo may initially undergo fragmentation, rather than cell death, in response to aneuploidy. We do not currently understand the mechanisms underlying the increased aneuploidy rates and frequent fragmentation observed in cleaving human embryos. However, we relate our data here to that in other organisms where genetic instability may be associated with unique epigenetic programs of preimplantation development [44] , [45] , [46] . Alternatively, generation of human embryonic aneuploidy may be related to the paternal contribution of the centrosome (and other spindle components) by the sperm for the first mitotic division [47] , [48] . Regardless of mechanism, it is likely that non-invasive assessment of development of human embryos as previously described [1] and further confirmed in the retrospective studies of clinical embryos will assist in the prediction of embryo viability [49] . Moreover, distinction between euploid and aneuploid embryos before transfer may contribute to improvements in IVF outcomes by potentially reducing the inadvertent transfer of embryos that would most likely result in embryonic lethality and spontaneous miscarriage. Sample source and procurement Approximately 85 two pronuclear and 25 cleavage-stage supernumerary human embryos from successful IVF cycles, subsequently donated for non-stem research, were obtained with written informed consent from the Stanford University RENEW Biobank. De-identification was performed according to the Stanford University Institutional Review Board-approved protocol #10466 entitled ‘The RENEW Biobank’ and the molecular analysis of the embryos was in compliance with institutional regulations. No protected health information was associated with individual embryos; ~25% of couples used donor gametes. Average maternal age was 33.5 years old and the most common cause of infertility was unexplained at 35.4% of couples. Human embryo thawing and culture Human embryos frozen at the zygotic or two pronuclear stage were thawed by a two-step rapid thawing protocol using Quinn’s Advantage Thaw Kit (CooperSurgical, Trumbull, CT) as previously described [1] . In brief, either cryostraws or vials were removed from the liquid nitrogen and exposed to air before incubating in a 37 °C water bath. Once thawed, embryos were transferred to a 0.5 mol l −1 sucrose solution for 10 min followed by a 0.2 mol l −1 sucrose solution for an additional 10 min. The embryos were then washed in Quinn’s Advantage Medium with Hepes (CooperSurgical) plus 5% serum protein substitute (CooperSurgical) and each transferred to a 60 μl microdrop of Quinn’s advantage cleavage medium (CooperSurgical) supplemented with 10% serum protein substitute under mineral oil (Sigma, St Louis, MO) and cultured at 37 °C with 6% CO 2 , 5% O 2 and 89% N 2 , standard human embryo culture conditions in accordance with current clinical IVF practice. Embryos were cultured in custom polystyrene petridishes with 25 individual microwells located in the centre to help track embryo identity during imaging and subsequent handling. Each microwell is 250 μm wide and 100 μm deep and accommodates a single developing embryo. To maintain group culture, all of the microwells share a common media drop, which is stabilized by an extruded ring. Small fiducial markers (letters and numbers) are located near the microwells for embryo identification. Time-lapse imaging and parameter analysis Embryo development was monitored using a custom-built miniature microscope system that can be placed on the shelf of a conventional incubator. The system consists of two inverted digital microscopes, each with light-emitting diode illumination, X10 Olympus objective, manual focus knob and 5 megapixel CMOS camera. The microscopes were modified for darkfield illumination by placing a darkfield aperture between the collimated white light-emitting diode and the condenser lens as previously described [1] . Images were taken at a 0.6 s exposure time every 5 min for up to 2 days (~30 h) until the majority of embryos reached the four-cell stage. The microscopes were connected to an external PC via USB cables that were passed through the rear access port of the incubator. A custom software program (written in C++) was used to control the microscopes, provide a user interface and save the images to file. After each experiment, images were compiled into a time-lapse movie with well-identification labels and timestamps that allowed manual measurement of the imaging parameters. The time interval for each cell cycle parameter was measured by three independent evaluators before the completion of the A-CGH and micronuclei analysis to ensure blinded parameter measurements. Automated tracking of cellular fragmentation The automated fragmentation detector is designed to seek geometrically coherent, yet short boundary segments throughout the image. As true cell boundary segments tend to be long, the detector considers the boundary segments <10 pixels in length to be those of fragments. First, boundary pixels are detected using a Hessian-based boundary detection, which provides boundary strength as well as orientation angle. Next, the boundary pixel locations and angles are analysed for coherence such that boundary pixels that form smooth continuous curves are grouped together as geometrically coherent segments. Finally, the grouped segments shorter than 10 pixels are classified as fragment boundary segments. Array-comparative genomic hybridization (A-CGH) Following imaging, the embryos were transferred to Acidified Tyrode’s Solution (Millipore) to remove the ZP and ZP-free embryos were disaggregated in Quinn’s advantage calcium and magnesium-free medium with Hepes plus 10% human albumin (CooperSurgical). Once disaggregated, each embryonic blastomere was washed three times in 10 μl drops of non-stick wash buffer and transferred to a sterile PCR tube. DNA extraction and preamplification was accomplished using the SurePlex Kit according to the manufacturer’s instructions (BlueGnome). In brief, the DNA was extracted from each sample as well as the reference sample with cell extraction enzyme at 75 °C for 10 min and the DNA was denatured and preamplified with PicoPlex pre-amp enzyme by a 95 °C hotstart for 2 min and 12 cycles of gradient PCR and then with PicoPlex amplification enzyme at 95 °C for 2 min and 14 cycles of 95 °C for 15 sec, 65 °C for 1 min and 75 °C for 1 min. Following whole genome amplification, each sample was fluorescently labelled with either Cy3 or Cy5 and hybridized to the BlueGnome CytoChip, which is a bacterial artificial chromosome array with >5,000 replicated clones designed to detect submicroscopic copy number variations, and covers ~30% of the human genome ( www.cytochip.com ). We chose A-CGH instead of alternatives for several reasons: First, A-CGH with the BlueGnome platform has now been validated in a large number of studies in reproductive clinics and genetic testing centres, including the detection of admixtures of chromosomally normal and aneuploid cell lines, single-cell analysis of embryos that were ultimately transferred and comparisons with other standard short tandem repeat (STR) methods [50] , [51] , [52] . Second, although the use of SNP arrays would also be very applicable, there is less information regarding the reliability of single-cell analysis and in many cases, inclusion of parental DNA is used to interpret many of the SNPs and eliminate potential complications such as allele drop out. Third, the genome coverage provided by A-CGH appeared sufficient to detect aneuploidies of every chromosome reliably. Scanned images were analysed and chromosomal copy number ratios quantified and reported using the CytoChip algorithm and BlueFuse software (BlueGnome). Threshold levels and whole chromosomal losses or gains were determined by three times the s.d., >±0.3 log 2 ratio call, or both as previously described [22] . Confocal imaging analysis and 3D modelling The ZP was removed by treatment with acidified Tyrode’s solution and ZP-free embryos were washed three times in PBS (Invitrogen, Carlsbad) with 0.1% bovine serum albumin (BSA; Sigma-Aldrich) and 0.1% Tween-20 (PBS-T; Sigma-Adrich), before fixation in 4% paraformaldehyde in PBS (USB Corp., Cleveland, OH) for 20 min at room temperature (RT). Once fixed, the embryos were washed three times in PBS-T to remove any residual fixative and stained with 1 μg ml −1 DAPI and 0.5 μg ml −1 MitoTracker Red CMXRos (Invitrogen) for 15 min at RT. For the visualization of CENP-A and LAMIN-B1, ZP-free embryos were fixed in 100% cold methanol at −20 °C for 15 min to preserve each epitope, washed and then permeabilized in 1% Triton X-100 (Sigma-Aldrich) for 1 h at RT. Following permeabilization, the embryos were washed three times in PBS-T and then blocked in 4% normal donkey serum (Jackson ImmunoReasearch Laboratories, Inc., West Grove, PA) in PBS-T overnight at 4 °C. The embryos were incubated with primary antibodies in PBS-T with 1% donkey serum sequentially for 1 h each at RT at the following dilutions: 1 μg ml −1 CENP-A (a kind gift from Ben Moree in Aaron Straight’s laboratory at Stanford University) and 1:1,000 rabbit LAMIN-B1 (Abcam; catalogue #ab16048). Primary signals were detected using the appropriate 488, 568 or 647-conjugated donkey Alexa Fluor secondary antibody (Invitrogen) at a 1:250 dilution at RT for 1 h in the dark. Immunofluorescence was visualized by sequential imaging, whereby the channel track was switched at the same focal plane each frame to avoid cross-contamination between channels set at 1 airy unit, using a Zeiss LSM510 Meta inverted laser scanning confocal microscope described here: http://nisms.stanford.edu/Equipment/LSM510Meta01v01.html . Confocal sections were captured at 1 mm intervals throughout the whole embryo and processed in ImageJ (NIH) for Z-stack imaging analysis. 3D reconstructions of embryos were accomplished with IMARIS (Bitplane). Fluorescent in situ hybridization FISH was performed by first incubating in a 1% tri-sodium citrate hypotonic buffer before fixation in Carnoy’s solution (3:1 ratio of methanol to glacial acetic acid) and then mounting on poly- L -lysine-treated slides (Fisher Scientific, Pittsburgh, PA) matured overnight at 60 °C. Hybridization to chromosome 18 (CEP 18/D18Z1/Spectrum Orange) and the Y-chromosome (CEP Y/DYZ1/Spectrum Aqua) was completed using fluorescently labelled DNA probes (Abbott Molecular, Des Plaines, IL) for 2 days in a 37 °C humidified chamber and positive signals were visualized by epifluorescent microscopy. FISH signals for chromosome 16 (CEP 16/D16Z3/Spectrum Green) and chromosome 21 (21q22.13-22.2/LSI 21/Spectrum Orange) were visualized with DAPI staining by confocal microscopy. Statistical analysis The individual parameter data is represented as the average ±s.d. and analysed for statistical significance ( P <0.05) using both one-way ANOVA with the Bonferonni multiple comparisons post-test and the non-parametric test, Kruskal–Wallis, with Dunn’s post-test. Fisher’s exact test was used to calculate the sensitivity and specificity of predicting aneuploidy with the parameters. How to cite this article: Chavez, S. L. et al . Dynamic blastomere behaviour reflects human embryo ploidy by the four-cell stage. Nat. Commun. 3:1251 doi: 10.1038/ncomms2249 (2012).